Using disorder to detect locally ordered electron nematics via hysteresis The interplay between charge, orbital and lattice degrees of freedom in correlated electron systems has resulted in many proposals for new electronic phases of matter. An electron nematic breaks the point group symmetry of the host crystal, often from C 6 or C 4 rotational symmetry to C 2 . Electron nematics have been reported in several condensed matter systems including cuprate- and iron arsenic-based high-temperature superconductors, and they have been proposed to exist in many other materials. However, the combination of reduced dimensionality and material disorder typically limits the spatial range over which electron nematic order persists, rendering its experimental detection extremely difficult. Despite the tantalizing possible connection between the phase and high-temperature superconductivity, there is surprisingly little guidance in the literature about how to detect the remaining disordered electron nematic. Here we propose two protocols for detecting disordered electron nematics in condensed matter systems using non-equilibrium methods. Signatures of electron nematic behaviour have been reported in a variety of materials, including Sr 3 Ru 2 O 7 (ref. 1 ), GaAs/Al x Ga 1− x As heterostructures in field [2] , [3] , and a subset of cuprate superconductors [4] , [5] , [6] , [7] , [8] , [9] , [10] such as YBa 2 Cu 3 O 6+ x (refs 5 , 6 , 7 ), and Bi 2 Sr 2 CaCu 2 O 8+ x (refs 8 , 9 , 10 ), as well as the iron arsenic based superconductor Ca(Fe 1− x Co x ) 2 As 2 (ref. 11 ). The state has been proposed to exist in many more systems, such as AlAs heterostructures, the Si(111) surface, elemental bismuth, and both single layer and bilayer graphene [4] , [12] , [13] , [14] . When an electron nematic forms, there is a preferred orientation to the electronic degrees of freedom, but the system remains invariant, under a rotation by π . In the case where the electron nematic breaks the in-plane C 4 (four-fold rotational) symmetry of the host crystal, there are two allowed orientations of the electron nematic, degenerate in energy. We therefore define a local nematic order parameter by σ =±1, corresponding to the two allowed orientations. ( Fig. 1 ). In a system with short-range interactions, the tendency for an electron nematic to form is described by a 'ferromagnetic coupling' J between these variables. In the absence of material disorder, the ground state is a long-range ordered electron nematic. 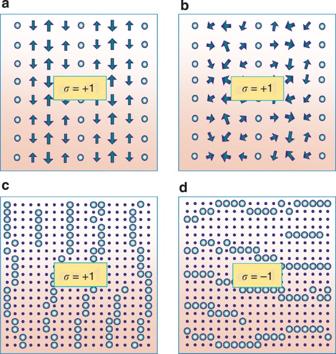Figure 1: Mapping of electron nematic orientations to Ising variables. (a) Fully ordered stripe state. Arrows represent spins residing within each crystalline unit cell, and circles represent charges. Because the charge component runs vertically, this is mapped toσ=+1.(b) Partially melted stripe state, with disordered spins. The charge component is the same as in part (a) mapping toσ=+1. (c) Nematic stripe state, oriented vertically. Large blue circles represent charge degrees of freedom. Small dark dots represent atomic positions with lower excess charge. A small concentration of dislocation defects in the charge-density wave are present, but the charge degrees of freedom maintain an overall orientation or nematicity. (d) Nematic stripe state, oriented horizontally. Disorder within any given region locally breaks the rotational symmetry of the host crystal, favouring one or the other nematic orientation, and thus presenting a random field on the nematic variable. Figure 1: Mapping of electron nematic orientations to Ising variables. ( a ) Fully ordered stripe state. Arrows represent spins residing within each crystalline unit cell, and circles represent charges. Because the charge component runs vertically, this is mapped to σ =+1. (b ) Partially melted stripe state, with disordered spins. The charge component is the same as in part ( a ) mapping to σ =+1. ( c ) Nematic stripe state, oriented vertically. Large blue circles represent charge degrees of freedom. Small dark dots represent atomic positions with lower excess charge. A small concentration of dislocation defects in the charge-density wave are present, but the charge degrees of freedom maintain an overall orientation or nematicity. ( d ) Nematic stripe state, oriented horizontally. Disorder within any given region locally breaks the rotational symmetry of the host crystal, favouring one or the other nematic orientation, and thus presenting a random field on the nematic variable. Full size image However, many of the materials mentioned above exhibit novel phases upon doping, a process which introduces intrinsic disorder [15] . Even in nominally clean materials, there remains a thermodynamically required concentration of defects at all non-zero temperatures. In any given region of such a sample, the pattern of dopant atoms or defects breaks rotational symmetry, and the resulting electric field gradients produce a locally preferred direction for the electron nematic. Because such disorder couples directly to the orientation of the electron nematic, we include its effects as a random field [16] : Here J || is an in-plane ferromagnetic coupling between nearest neighbour (Ising) nematic variables σ , J ⊥ represents the coupling between nematic variables in neighbouring planes, and the random field h i is chosen from a gaussian probability distribution centred about zero, with width Δ , which we will call 'random field strength'. The effects of material disorder can also introduce local energy-density disorder in the form of randomness in these couplings, but as long as the randomness does not introduce a finite density of frustrated plaquettes, the universal non-equilibrium behaviour is described by equation (1) [17] . (See the Methods section for more details.) In the limit of zero random field strength, the model has a finite-temperature continuous phase transition for dimension d ≥2. 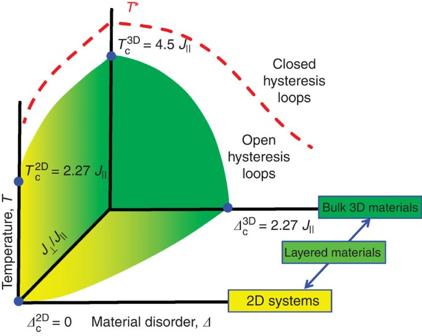Figure 2: Schematic phase diagram of electron nematics from two to three dimensions. The solid region (yellow to green) denotes the ordered phase, with yellow corresponding to 2D systems, and green corresponding to 3D systems. In two dimensions (J⊥/J||=0), appropriate to graphene and interfaces such as surfaces and quantum Hall systems, the critical disorder strength isΔc2D=0, and consequently in any real 2D system the electron nematic is disordered. An ordered electron nematic is possible in 2D only, when the material has zero defects. In bulk materials, there is a finite critical disorder strength, below which the system shows an ordered nematic at low temperature. Strongly layered materials such as cuprate superconductors are closer to the 2D regime than the 3D limit, and thus have a smaller region where the electron nematic may be long-range ordered than in the fully 3D limit. Dashed lines indicate the disorder dependent crossover temperatureT*(Δ,Ω) marking a change in behaviour of hysteresis loops in electronic nematicity versus applied orienting field. At high temperatures, hysteresis is not observable, and the system shows the equilibrium paramagnetic behaviour as an external orienting field is changed. For a given field, sweep amplitudeHoand sweep rateΩat which the external field is changed,T*(Δ,Ω) marks the crossover temperature below which the system can no longer equilibrate, marked by open hysteresis loops. However, as shown schematically in Figure 2 , for any finite random field strength, long-range electron nematic order is forbidden in two-dimensional systems like graphene, surfaces and two-dimensional electron gases. Even in strongly layered materials (such as certain transition metal oxides), or highly anisotropic bulk materials (such as bismuth), the electron nematic may be forbidden to arise because of quenched disorder. However even in the disordered phase, the nematic domains will have a large characteristic size, if the disorder is sufficiently weak, and they will be correspondingly important for the macroscopic physics. Figure 2: Schematic phase diagram of electron nematics from two to three dimensions. The solid region (yellow to green) denotes the ordered phase, with yellow corresponding to 2D systems, and green corresponding to 3D systems. In two dimensions ( J ⊥ / J || =0), appropriate to graphene and interfaces such as surfaces and quantum Hall systems, the critical disorder strength is Δ c 2D =0, and consequently in any real 2D system the electron nematic is disordered. An ordered electron nematic is possible in 2D only, when the material has zero defects. In bulk materials, there is a finite critical disorder strength, below which the system shows an ordered nematic at low temperature. Strongly layered materials such as cuprate superconductors are closer to the 2D regime than the 3D limit, and thus have a smaller region where the electron nematic may be long-range ordered than in the fully 3D limit. Dashed lines indicate the disorder dependent crossover temperature T *( Δ , Ω ) marking a change in behaviour of hysteresis loops in electronic nematicity versus applied orienting field. At high temperatures, hysteresis is not observable, and the system shows the equilibrium paramagnetic behaviour as an external orienting field is changed. For a given field, sweep amplitude H o and sweep rate Ω at which the external field is changed, T *( Δ , Ω ) marks the crossover temperature below which the system can no longer equilibrate, marked by open hysteresis loops. Full size image It is therefore crucial to understand how to detect local electronic nematic behaviour, especially in the disordered phase. Significant progress has recently been made via scanning tunnelling microscopy [9] , [10] , [18] . However, probes limited to the surface cannot address the question of whether similar physics arises in the bulk of the material. Furthermore, such imaging techniques are not available for two-dimensional electron gases. For this reason, it is vital to develop new ways to detect disordered electron nematics using bulk macroscopic measurement techniques. The methods described here can be applied to macroscopic measurements as well as to local probes. The degree of electron nematic order in the system is described by the orientational order parameter, N =(1/ V )∑ i σ i where V is the number of sites in the system. The order parameter (nematicity) is N =1 when all nematic domains are aligned along, for example, the x axis, and it is N =−1 when all domains align along the y axis. The external field h represents any applied field which breaks orientational symmetry. An example is an applied magnetic field which maps to the orientational field as , where χ x y is proportional to the diamagnetic anisotropy. See Tables 1 and 2 for experimentally accessible orienting fields, as well as experimental measures of electron nematic order. Table 1 Orienting fields. Full size table Table 2 Order parameters. Full size table In this paper, we propose two non-equilibrium protocols for detecting electron nematicity via hysteresis in nematicity versus applied orienting field ( Tables 1 and 2 ). The first is an extension of the usual field-cooling protocol for ferromagnets to the case of nematics (with some subtleties explained below), whereas the second is an entirely new protocol for distinguishing nematics from magnetic domains. Nonequilibrium protocols for electron nematicity Below a crossover temperature T * (denoted by the red dashed line in Fig. 2 ), the macroscopic nematic order exhibits 'hysteresis' with respect to the applied orienting field, signalling proximity to the ordered phase. Unfortunately, hysteresis loops are closed in thermal equilibrium. Fortunately, equilibrium is hard to achieve in this model. Because the phase transition is controlled by a zero-temperature fixed point, the energy barriers to equilibration diverge at the critical disorder as temperature decreases in the thermodynamic limit [19] . In fact, for any finite sweep rate Ω of the externally applied orienting field, hysteresis loops remain open (and the system is out of equilibrium) for | H |< H neq ( T ,Ω). Therefore, for any given sweep rate Ω and field sweep amplitude H o there exists a crossover temperature, as shown in Figure 2 , below which the hysteresis loops will be open over the entire range − H o to H o , indicating the presence of a disordered nematic. In the case of the (low-temperature) saturation hysteresis loop, the sign of the order parameter does not change until the coercive field strength is achieved. However, the coercive field strength is a nonuniversal property which varies from material to material. In cases where the low-temperature coercive-field strength is either unknown a priori or unachievable, it is important to design new methods capable of revealing the hysteresis even at low strength of the orienting field. Extension of field-cooling protocol We, therefore, focus here on universal properties of hysteresis, applicable to disordered electron nematics in any system. The first protocol we propose is an extension of the idea of field-cooling ferromagnets (as used, for example, to prepare commercial permanent magnets) [20] to the case of disordered nematics in condensed matter systems. Using a magnetic field as orienting field and transport anisotropy as a measure of nematic order, the method we propose is as follows (Steps 1–4 are shown schematically in Fig. 3a ): Start from a high-temperature equilibrium configuration (Step 1 in the figure). Apply a magnetic field parallel to the x axis, (Step 2 in the figure). Cool in field (Step 3 in the figure). Turn off the applied field (Step 4 in the figure). Measure the nematic order parameter via, for example, ρ xx − ρ yy . Zero-field warm the sample to the starting high temperature. Apply the magnetic field parallel to the y axis, and field cool to the same temperature as before. Turn off the applied field. Measure again the macroscopic anisotropy, for example, ρ xx − ρ yy . Our prediction is that ρ xx − ρ yy will switch sign under this protocol, if the system has nematic domains which locally break C 4 symmetry to C 2 symmetry. If hysteresis is detected, several more extensive hysteresis tests can be applied to gain more information about the nature of the interactions, as discussed in the Discussion Section. (There are slight modifications needed for the case of breaking a C 6 symmetry down to C 2 symmetry.) 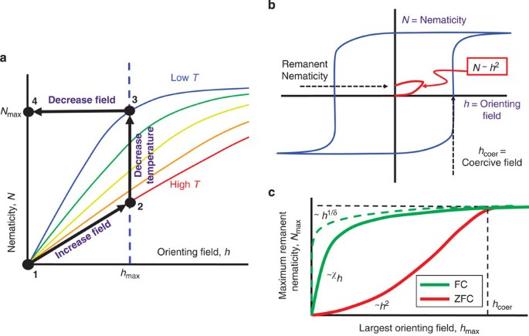Figure 3: Remanent nematicity under different protocols. (a) Field-cooling method to maximize remanent nematicity. Steps 1–4 are described in the text. (b) The outer loop (thin blue line) is the saturation hysteresis loop at low temperatue, accessible only if the coercive field strength is attainable. The smaller curve (thick red line) shows the response upon application of a weak orienting field, starting from a zero field cooled configuration. With zero field cooling, the maximum achievable remanent nematicity for a given maximum applied field is bounded by the Rayleigh law, and is therefore weak. (c) Comparison of the maximum remanent nematicity in the field cooling (solid green line) and zero-field cooling (solid red line) methods, for the same maximum applied orienting field. The green dotted line is the asymptotic behaviour in the field cooling case, as the temperature is lowered to the critical point. The maximum remanent nematicity is significantly higher in the field-cooling method (by one or more powers ofh), as compared with the zero field cooling case, especially for weak applied fields. Figure 3: Remanent nematicity under different protocols. ( a ) Field-cooling method to maximize remanent nematicity. Steps 1–4 are described in the text. ( b ) The outer loop (thin blue line) is the saturation hysteresis loop at low temperatue, accessible only if the coercive field strength is attainable. The smaller curve (thick red line) shows the response upon application of a weak orienting field, starting from a zero field cooled configuration. With zero field cooling, the maximum achievable remanent nematicity for a given maximum applied field is bounded by the Rayleigh law, and is therefore weak. ( c ) Comparison of the maximum remanent nematicity in the field cooling (solid green line) and zero-field cooling (solid red line) methods, for the same maximum applied orienting field. The green dotted line is the asymptotic behaviour in the field cooling case, as the temperature is lowered to the critical point. The maximum remanent nematicity is significantly higher in the field-cooling method (by one or more powers of h ), as compared with the zero field cooling case, especially for weak applied fields. Full size image In Figure 3 we show the maximum possible remanent nematicity, both for the method described here, and for a remanent nematicity obtained after zero-field cooling and then training in field. One can see that at low applied fields, the nematic order parameter is enhanced by at least one power of h for field cooling over zero-field cooling, and it is enhanced even more near criticality (see below). A major advantage to this protocol is the ability to detect nematicity even with weak applied fields, that is, the principles apply even in cases where the coercive field strength is either unknown or inaccessible experimentally. Furthermore, because we have focused on universal behaviour, the principles apply to disordered electron nematics in any condensed matter system, with any combination of applied orienting field and measure of nematicity. There are two important things to notice about Figure 3 . First, starting from the (disordered) thermal equilibrium configuration, the nematicity rises as N χh upon application of a weak field in thermal equilibrium, with a susceptibility that diverges at the critical point as χ h 1/δ−1 , corresponding to the dotted green line in Figure 3c . Because the model (equation 1) has a wide critical region [17] , the susceptibility is large in a wide region of parameters, leading to a rapid increase of N as h is applied, N h 1/δ . For the finite disorder critical point of the three-dimensional random field Ising model (RFIM, equation 1), βδ =1.81±0.32 and β =0.035±0.028 (ref. 21 ). Although the uncertainty on 1/ δ itself is high, the value of 1/ δ is low (it is roughly 1/ δ =0.019±0.16), so that when following the equilibrium (paramagnetic) magnetization curves, the nematicity rises dramatically (as N h 0.019 ) as a weak field is applied. Materials which are layered will also have a regime of two-dimensional scaling, before reaching the 3D-scaling regime [22] . For 2D-RFIM scaling, 1/ δ goes to zero, and the rise in nematicity with weak applied field is even faster. Second, the nematicity increases as the temperature is lowered in weak applied field ( Fig. 3a ). The low-field slope of the equilibrium nematicity versus applied orienting curve is controlled by the susceptibility of the RFIM, which increases as | T − T c | β (1− δ ) near the critical point. Note that application of a field reduces the barriers to equilibration, so that the magnetization tracks the equilibrium magnetization curves throughout much of the field-cooling process. Once the system is cooled below the temperature T *( Δ ) at which it falls out of equilibrium (that is, when the nematicity plateaus), the orienting field should be turned off (Step 4), and the remanent magnetization measured. This method is sensitive to locally oriented objects of any type, including orientational defects in a lattice as well as magnetic domains. Many forms of magnetic broken rotational symmetry can be more easily detected by other means, such as net magnetization, neutron scattering, or superconducting quantum interference device magnetometry. However, some forms of magnetism are more subtle [23] , [24] , such as those which break time-reversal symmetry without breaking the translational symmetry of the host crystal. Note that the response of magnetic domains to our method will not directly induce a sign change in ρ xx − ρ yy . Rather, the response of magnetic domains to this protocol causes M y ρ xz − ρ zx and M x ρ yz − ρ zy to exchange values. Furthermore, while magnetoresistance is a standard phenomenon, it is not generically hysteretic. On the other hand, effects such as magnetostriction can couple in-plane magnetic moments to in-plane lattice distortions, inducing a (weak) secondary response in ρ xx − ρ yy . Distinguishing nematics from magnetic domains Nematic domains can be distinguished from subtle time-reversal symmetry breaking by extending the method as follows ( Fig. 4 ). After following steps (1)-(4) above with, for example, to achieve a (non-equilibrium) field-cooled configuration, then apply step (5a): ramp the field back up to its maximum value and measure ρ xx − ρ yy in field. Next, turn off the field, raise the temperature, and follow steps (1)–(4) again, also with . At this point, apply step (5b): ramp the field to the same maximum magnitude, but in the opposite direction (that is, ) and measure ρ xx − ρ yy in field. Magnetic domains respond quite differently in the two cases, whereas the nematic order parameter responds exactly the same way in both extended versions. Furthermore, in the extended protocol, magnetic order parameters respond smoothly through H =0, whereas nematic domains show a kink at H =0 for slow enough sweep rates. The following inequalities also apply: where N (4) and M (4) represent, for example, the nematicity and magnetization, respectively, at the end of step 4. These techniques can be used to illuminate the connection between electron nematicity and high temperature superconductivity, as well as to address the question of whether the phase is present in the wide variety of materials for which this exotic electronic phase of matter has been proposed yet remains undetected. Furthermore, rather than requiring ultraclean materials, the methods described here are only helped by the disorder which is surely present in all macroscopic samples. 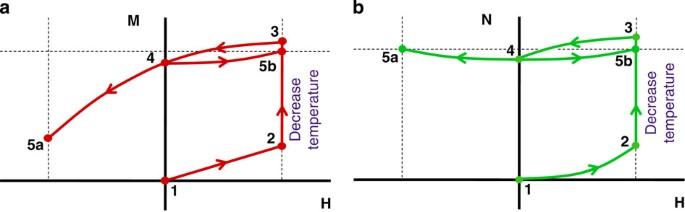Figure 4: Extended protocol. (a) Behaviour of magnetic domains under extended protocol (see text for description). Magnetic domains respond very differently when following steps (1)–(5a) versus following steps (1)–(5b). (b) Behaviour of nematic domains under extended protocol (see text for description). In sharp contrast to magnetic domains, nematic domains respond in the same way whether following steps (1)–(5a) or steps (1)–(5b). Figure 4: Extended protocol. ( a ) Behaviour of magnetic domains under extended protocol (see text for description). Magnetic domains respond very differently when following steps (1)–(5a) versus following steps (1)–(5b). ( b ) Behaviour of nematic domains under extended protocol (see text for description). In sharp contrast to magnetic domains, nematic domains respond in the same way whether following steps (1)–(5a) or steps (1)–(5b). Full size image The protocols described above are tuned to the case where the original crystal structure has two equivalent axes, say a and b , along which nematicity may develop. Then, upon entering an electron nematic phase, the symmetry between a and b directions is spontaneously broken. A good candidate material in the cuprates for the proposed protocols is BSCCO. Although there is a supermodulation present, the lattice modulation is along the diagonal to the copper–oxygen bonds within the Cu-O planes, and it does not couple to the nematic director. The cuprate superconductor YBCO has an explicitly broken rotational symmetry due to the Cu–O chains which reside between planes. This effect can be captured within our model as a static, constant internal orienting field, h o . Upon applying any of the protocols here to YBCO, care must be taken to remember that the system starts with an intrinsic orienting field h o . It may be possible to counteract this intrinsic crystalline effect by application of an appropriately chosen external orienting field h e , such that h o + h e =0 and the total orienting field cancels. For the cuprate family LSCO, such a cancellation is not possible, since the effective internal field changes sign from one Cu–O plane to the next. This can be captured within equation (1) with an intrinsic orienting field h o which changes sign from plane to plane, however such a model has not yet been studied in detail. Other good candidate systems include those for which electron nematicity is predicted to arise from valley degeneracy breaking of otherwise four-fold symmetric valleys, such as in AlAs heterostructures and the Si(111) surface [12] . Note that in contrast to AlAs heterostructures, where the valley symmetry is discrete and its breaking can be described by an Ising order parameter, in GaAs/Al x Ga 1− x As heterostructures the development of the nematic has been linked to an XY model (rather than Ising model), in a weak symmetry-breaking field [25] , [26] , [27] . If the protocols described above give a positive result, several more extensive hysteresis tests can be applied [28] : For example, the model predicts that subloops should close at low temperature, and also exhibit return point memory. Two different subloops between the same extremal fields but with 'different histories' should be incongruent if the domains interact, whereas a collection of independent hysteretic switchers yields congruent subloops. Hysteresis can also be explored as a function of angle within the plane. Because if an applied magnetic field is rotated within the xy plane, the nematic order parameter responds with a period which is half that of a magnetic order parameter. Mapping electron nematics to ising variables with disorder One way that electron nematics arise is by melting a stripe phase [29] as shown in Figure 1 . (For some other ways, see for example, ref. 30 .) A fully ordered stripe phase is a unidirectional, interleaved charge and spin density wave ( Fig. 1a ). As temperature or quantum fluctuations are increased in such a system, spin order is generally lost before charge order ( Fig. 1b ). As temperature or quantum fluctuations increase, dislocations in the charge stripe order lead to a nematic phase. ( Fig. 1c ). In each of these examples, there is orientational order present in the charge degrees of freedom, and it is this directionality which locks to the crystalline direction. Figure 1a–c have the charge component of the stripes running vertically, mapping to Ising variable σ =+1. (See equation (1) in the main text.) Figure 1d has the charge orientation running horizontally, mapping to Ising variable σ =−1. Effects of material disorder Thermodynamics requires that in any given material, there is a finite concentration of defects, driven by the entropy of mixing. Although the effects of disorder may have several different manifestations in the microscopic physics, at the level of an order parameter description, there are two classes of disorder: random field disorder, and local energy-density disorder (also known as random T c disorder) [31] . In equation (1) of the main text, we have introduced the effects of material disorder (such as dopant atoms) in the form of a random field on the Ising variable. This is because in general, the local pattern of disorder induced by material defects breaks rotational symmetry, and, therefore, by symmetry, it must couple linearly to the order parameter. Material disorder can also induce the second type of disorder at the order-parameter level, namely local energy-density disorder. This may directly enter the model as randomness in the couplings J ij , or as randomness in the local strength of the nematic order parameter, which may then be subsumed into randomness in the couplings J ij . As long as the mean value of the random couplings remains positive, the universal non-equilibrium behaviour of this type of random bond Ising model is the same as that of the random field Ising model for non-equilibrium phenomena, because application of an orientating field explicitly breaks the σ =±1 symmetry [32] . Furthermore, if both types of disorder are present, the universal equilibrium behaviour is also that of the random field Ising model. If the disorder is purely of the local energy-density type (such as random bond disorder with no random field disorder), then in the equilibrium phase diagram, the ordered phase becomes more stable. In particular, the ordered phase remains stable against weak random bond disorder in two dimensions. However, sufficiently strong disorder of either type (random bond or random field) can lead to the destruction of the long-ranged nematic phase, in which case the protocols described here can be used to test for local nematic behaviour. The behaviour of the system under our protocols is controlled by the non-equilibrium behaviour, and the universal non-equilibrium properties in the presence of either type of disorder are described by equation (1) in the main text. Phase transition line in the T =0 plane As shown in Figure 1 , at zero temperature, there is a disorder-driven phase transition from the ordered nematic phase into a disordered phase. In three dimensions, this obtains at a critical disorder strength of Δ c 3D = 2.27 J ∥ [33] ), whereas in two dimensions the critical disorder strength is Δ c 2D = 0 (ref. 34 ), and there can be no nematic phase in a 2D system with any finite material disorder strength. In a strongly layered system with J ⊥ / J ∥ ≪ 1 (ref. 22 ), the critical disorder strength is a logarithmic function of interlayer coupling: where σ≈0.29 (ref. 35 ), and c o is a constant of order 1(ref. 22 ). Near the 3D limit, 1− J ⊥ / J ∥ ≪ 1 and the critical disorder strength is a linear function of interlayer coupling [22] : where c 1 is a constant of order 1. How to cite this article: Carlson, E.W. & Dahmen, K.A. Using disorder to detect locally ordered electron nematics via hysteresis. Nat. Commun. 2:379 doi: 10.1038/ncomms1375 (2011).